A fully genetically encoded protein architecture for optical control of peptide ligand concentration Ion channels are among the most important proteins in biology, regulating the activity of excitable cells and changing in diseases. Ideally it would be possible to actuate endogenous ion channels, in a temporally precise and reversible manner, and without requiring chemical cofactors. Here we present a modular protein architecture for fully genetically encoded, light-modulated control of ligands that modulate ion channels of a targeted cell. Our reagent, which we call a lumitoxin, combines a photoswitch and an ion channel-blocking peptide toxin. Illumination causes the photoswitch to unfold, lowering the toxin’s local concentration near the cell surface, and enabling the ion channel to function. We explore lumitoxin modularity by showing operation with peptide toxins that target different voltage-dependent K + channels. The lumitoxin architecture may represent a new kind of modular protein-engineering strategy for designing light-activated proteins, and thus may enable development of novel tools for modulating cellular physiology. Ion channels govern cellular signaling and computation, in neurons and neural compartments as well as other excitable cell classes, and are significant drug targets for a variety of disorders [1] , [2] . Ideally, one could genetically target ion channels for perturbation to assess their causal contribution to complex systems. Earlier studies have approached this problem by several kinds of innovation. For example, one line of inquiry has resulted in genetically encoded membrane-targeted peptide toxins that can be expressed in cell types of interest. Peptide toxins comprise a broad class of genetically encoded ion channel modulators from venomous animals that are capable of recognizing targets from every major ion channel family, with extraordinary specificity [3] , [4] , [5] , [6] , [7] , [8] . These reagents function without requiring exogenously supplied chemicals, and are inducible and reversible over timescales of hours to days [9] , [10] , [11] , [12] , and have been shown to function in mammalian brain in vivo . A second line of inquiry has utilized light-responsive chemical modulators that are anchored to specific sites engineered into ion channels (for example, SPARK, LiGluR and HyLighter) [13] , [14] , [15] , [16] , [17] , [18] , [19] , and thus are capable of fast induction and reversal with light. They incorporate exogenously supplied engineered chemicals, which bind to engineered sites on targeted ion channels. The first technology is fully genetically encoded but not light-modulatable; the second technology is rapidly light-modulatable but not genetically encoded. Here we devise a novel protein architecture capable of modulating endogenous ion channels, but which is both fully genetically encoded, and actuatable by light. We accordingly here adapt three different technology building blocks in a novel protein architecture to yield a fully genetically encoded reagent that can actuate endogenous voltage-gated K + (Kv) channels with light. We create a fusion protein containing a peptide toxin as the ion channel ligand and a light-oxygen-voltage (LOV) domain photoswitch tethered to the cell membrane. We hypothesize that upon illumination, conformational changes in the LOV domain lower the local concentration of the peptide toxin near the cell surface, and thus enables the ion channel target’s functionality in response to light. We develop a quantitative theory for the function of these ‘lumitoxins’ and characterize the biophysical properties of an α-dendrotoxin-bearing lumitoxin modulating Kv channels expressed in mammalian cells. We create a library of lumitoxins made of mutated peptide toxin variants to illustrate the tunability of our system. Finally, we establish modularity of the lumitoxin protein architecture by creating several lumitoxins containing genetically encoded K + channel blockers, which upon illumination will disinhibit different subclasses of Kv channels. Our modular, simple architecture for light-controlled protein ligand concentration may provide a platform for rapidly making new libraries of novel light-actuatable protein ligands that are genetically targetable. A theory for light-actuated tethered protein ligands Owing to the great structural and functional knowledge about potassium channels [20] , [21] , we focused on Kv channels for this study. One exemplar implementation of the lumitoxin architecture is to express a fusion protein that contains a Kv channel-specific peptide toxin (for example, α-Dendrotoxin, αDTX), and a photoreceptor domain [22] , [23] (for example, LOV2-Jα), targeted to the secretion pathway and anchored to the extracellular side of the cell membrane ( Fig. 1a ). To acquire some intuition about potential mechanisms of operation of such reagents, we implemented a simplified tethered-particle motion model of this hypothetical fusion protein and simulated its diffusive behaviour to gain insight into the characteristic parameters. Our simulation predicts that the number of peptide collisions with the cell surface is decreased as the tether length is increased, the computational analogue to the unfolding of the Jα helix. Specifically, by inspecting the probability distribution in the x–z plane (that is, looking at the lumitoxin from the side as in Fig. 1a ) we get an appreciation of the changes in the mean peptide localization. Shown are the simulation results for a six-membered and a 27-membered membrane linker (Fig. 1b , upper left and lower left panels, respectively). The distribution difference demonstrates that after unfolding of the Jα helix, it is more likely to find the peptide 6 nm away from the membrane plane; the local concentration close to the peptide toxin’s binding site on a membrane-bound ion channel would accordingly be greatly reduced ( Fig. 1b , right panel). 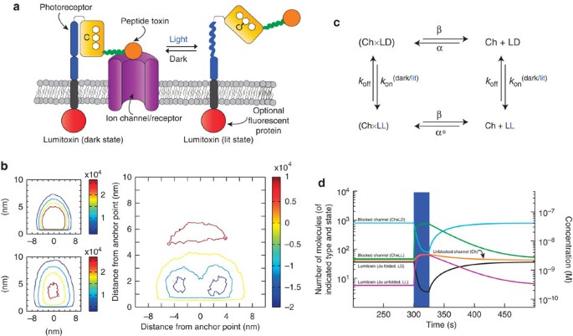Figure 1:A theoretical framework for light-actuated tethered protein ligands. (a) Architecture of fusion protein containing a membrane-anchored (PDGF-R, black) photoreceptor AsLOV2 (yellow; ‘C’ indicates the location of key cysteine, and molecular structure schematically represents flavin)/Jα (blue) connected to a peptide toxin (orange) via a flexible linker (green wiggly line), optionally equipped with a fluorophore (red sphere). (b) Tethered-particle motion model: location probability of encountering the peptide domain projected on thex–zplane (that is, where the membrane is thex–yplane) for a short (6/26, upper left panel) versus longer membrane tether (27/26, lower left panel). Numbers before and after the ‘/’ indicate length, in amino acids, of the blue and green linkers, respectively. The difference (right panel) indicates that increasing the tether length decreases the peptide concentration close to the cell surface. (c) A model describing the binding equilibrium of a hypothetical protein adopting two different states (dark and lit) differing in biological activity (high affinity and low affinity)—LD and LL, respectively, to an ion channel (Ch). (d) Simulation of the dynamic response of the model depicted in (c) to illumination, indicated by blue bar (see legends). See methods for model parameters. Figure 1: A theoretical framework for light-actuated tethered protein ligands. ( a ) Architecture of fusion protein containing a membrane-anchored (PDGF-R, black) photoreceptor AsLOV2 (yellow; ‘C’ indicates the location of key cysteine, and molecular structure schematically represents flavin)/Jα (blue) connected to a peptide toxin (orange) via a flexible linker (green wiggly line), optionally equipped with a fluorophore (red sphere). ( b ) Tethered-particle motion model: location probability of encountering the peptide domain projected on the x–z plane (that is, where the membrane is the x–y plane) for a short (6/26, upper left panel) versus longer membrane tether (27/26, lower left panel). Numbers before and after the ‘/’ indicate length, in amino acids, of the blue and green linkers, respectively. The difference (right panel) indicates that increasing the tether length decreases the peptide concentration close to the cell surface. ( c ) A model describing the binding equilibrium of a hypothetical protein adopting two different states (dark and lit) differing in biological activity (high affinity and low affinity)—LD and LL, respectively, to an ion channel (Ch). ( d ) Simulation of the dynamic response of the model depicted in ( c ) to illumination, indicated by blue bar (see legends). See methods for model parameters. Full size image The effect of this apparent dilution can be understood if we consider an equilibrium system in which a lumitoxin can adopt two different states, Lit (LL) or Dark (LD) ( Fig. 1c ). Here the lit-state of the membrane-tethered peptide toxin has a lower local concentration near the cell surface, resulting in a decreased apparent association rate constant ( α *) for binding to the channel (Ch) and then blocking it (Ch × LL or Ch × LD). As approximations, we assume that the lumitoxin and channel are expressed to similar levels, and further assume that the dynamics of light-dependent conformational changes in the LOV-Jα photoreceptor are independent of the peptide toxin/channel binding equilibrium. We found that when using published values for the binding of α-DTX to Kv [24] , [25] and the light-dependent transitions of an isolated LOV2-Jα domain from Avena sativa [26] , [27] (see Methods for details), the system equilibrates with most ion channels (>90%) being occupied by a peptide toxin—that is, most Kv channels are blocked by the tethered αDTX in the dark state ( Fig. 1d , compare cyan (blocked channel) and orange (unblocked channel) lines). Illumination leads to a rapid increase in unblocked ion channels, followed by a somewhat slower re-blocking of those channels when illumination ceases. On the basis of our simulations we predict that a synthetic fusion protein, as we described above, will react to illumination with reasonably fast response times (s) and will allow fully reversible repeated activation/deactivation cycles. Lumitoxins mediate optical modulation of cellular K + current We synthesized a gene coding for a lumitoxin that contained Dendroaspis angusticeps αDTX, which specifically binds to Kv1.1 and Kv1.2 channels, connected to the A. sativa LOV2-Jα domain (AsLOV2) via a 26-residue flexible linker. This fusion protein was targeted for the secretory pathway using a cleavable signal peptide and was anchored to the extracellular side of the cell membrane by a single-pass transmembrane domain derived from the human platelet-derived growth factor receptor (PDGF-R). We expressed αDTX–lumitoxins in cultured PC12 cells co-transfected with Kv1.2, and saw healthy expression ( Fig. 2a ), as might be expected, given that both AsLOV2-containing proteins and peptide toxins had previously been shown separately to express in mammalian cells. Whole-cell patch clamp recordings showed characteristic baseline voltage-dependent K + currents in a cell expressing αDTX–lumitoxins ( Fig. 2b , left panel). Illumination of the same cell with modest levels (500 μW mm −2 ) of blue (455 nm) light increased the whole-cell K + current approximately twofold within seconds ( Fig. 2c , orange circles and Fig. 2b , middle panel). After cessation of illumination, the whole-cell K + current recovered to pre-illumination levels within 2 min ( Fig. 2b , right panel). 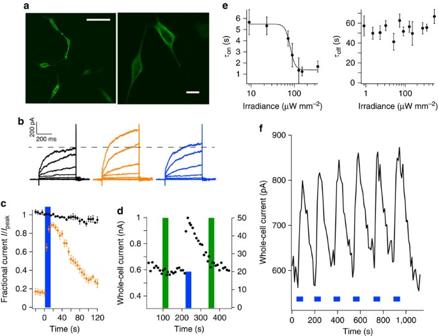Figure 2:Lumitoxins mediate light actuation of specific Kv channels. (a) PC12 cells expressing FLAG-tagged lumitoxins containing AsLOV2 and α-Dendrotoxin (αDTX), here denoted dendrolumitoxin. Cells are fixed and stained with α-FLAG/Alexa 488. Scale bar, 100 μm (left panel), 20 μm (right panel). (b) Whole-cell K+currents before (black), during (orange) and after (blue) illumination with 500 μW mm−2blue (455 nm) light (colour and power used throughout, unless otherwise indicated). Holding voltage −80 mV, depolarization voltages increasing in increments of 10 mV to +50 mV. (c) Normalized whole-cell K+current modulation (that is, current divided by maximum observed currentIpeak) in response to blue-light illumination (blue bar) recorded in PC12 cells co-expressing dendrolumitoxin with Kv1.2 (orange) or Shaker (black). Plotted throughout is the mean plus or minus s.e.m.,n=3 cells. (d) Dendrolumitoxin modulation of Kv1.2 responds to blue (455 nm, blue bar) but not green (530 nm, green bars) light. (e) Dependence of apparentτonand apparentτoffof whole-cell Kv1.2 current modulation (that is, curves plotted as inc) on irradiance.n=2–4 cells each point. (f) Repeated modulation of whole-cell Kv1.2 current with illumination (blue bars). Figure 2: Lumitoxins mediate light actuation of specific Kv channels. ( a ) PC12 cells expressing FLAG-tagged lumitoxins containing AsLOV2 and α-Dendrotoxin (αDTX), here denoted dendrolumitoxin. Cells are fixed and stained with α-FLAG/Alexa 488. Scale bar, 100 μm (left panel), 20 μm (right panel). ( b ) Whole-cell K + currents before (black), during (orange) and after (blue) illumination with 500 μW mm −2 blue (455 nm) light (colour and power used throughout, unless otherwise indicated). Holding voltage −80 mV, depolarization voltages increasing in increments of 10 mV to +50 mV. ( c ) Normalized whole-cell K + current modulation (that is, current divided by maximum observed current I peak ) in response to blue-light illumination (blue bar) recorded in PC12 cells co-expressing dendrolumitoxin with Kv1.2 (orange) or Shaker (black). Plotted throughout is the mean plus or minus s.e.m., n =3 cells. ( d ) Dendrolumitoxin modulation of Kv1.2 responds to blue (455 nm, blue bar) but not green (530 nm, green bars) light. ( e ) Dependence of apparent τ on and apparent τ off of whole-cell Kv1.2 current modulation (that is, curves plotted as in c ) on irradiance. n =2–4 cells each point. ( f ) Repeated modulation of whole-cell Kv1.2 current with illumination (blue bars). Full size image As predicted by our model ( Fig. 1 ), the majority of ion channels were blocked in the dark state, as judged by the baseline K + currents recorded in cells co-expressing both αDTX–lumitoxin and Kv1.2 versus cells expressing Kv1.2 alone (mean current at +50 mV: 40±12 pA/pF versus 206±24 pA/pF, P <0.0001 two-tailed Student’s t -test, n =7–20). Furthermore, as predicted by our model, the whole-cell K + current rose within seconds and then, post illumination, attenuated back to baseline somewhat more slowly, but completely ( Fig. 2c , orange circles). An important aspect of the utility of peptide toxins in physiology and neuroscience is their excellent specificity; they can differentiate between subfamilies of closely related ion channels and receptors. To test whether the observed light-dependent current increase was ion channel-specific, we co-expressed the Shaker channel and αDTX–lumitoxin in the same cell. Kv1.2 and Shaker are similar in many aspects, but differ in their sensitivity to αDTX; αDTX binds to Kv1.2 with picomolar affinity, while its affinity for Shaker is very low (micromolar) [25] . As expected, illumination did not alter whole-cell K + current in cells that co-expressed Shaker and αDTX-lumitoxin, demonstrating that peptide toxins embedded within lumitoxins maintain their binding specificity ( Fig. 2c , black circles). Neither were the properties of the AsLOV2 domain overtly perturbed by embedding within a lumitoxin, as current modulation was dependent on blue light, and was not affected by green light ( Fig. 2d ). We measured the time constant for light-driven lumitoxin effect—that is, the time constant constant by which the Jα helix unfolds and presumably lowers the local αDTX concentration near the cell surface—leading to an increase in available Kv1.2 channels. We found the time constant to be a function of irradiance, consistent with Jα helix unfolding being dependent on photon absorption. The apparent half-maximum time constant is achieved at 80 μW mm −2 ( Fig. 2e , left panel). Thus, note that K + current could be modulated by non-damaging, relatively low light intensities. On the other hand, the post-illumination recovery of K + current to pre-illumination baseline, associated with an increase in αDTX concentration close to the membrane-bound ion channel and increased block of Kv1.2, solely depends on the spontaneous dark-state refolding of LOV2-Jα and is thus expected to be independent of irradiance, which we confirmed experimentally ( Fig. 2e , right panel). Repeated stimulation with blue light demonstrates that αDTX–lumitoxins are able to carry out consecutive K + current modulations and are not undergoing destructive conformational changes ( Fig. 2f ). The lumitoxin architecture enables rational protein design We assessed the tunability of the lumitoxin architecture by utilizing a family of mutated αDTX variants, which are known to possess altered affinity towards Kv1.2. High-affinity binding of αDTX depends crucially on the peptide residues K5 and L9, and changing them to alanine decreases the binding affinity by three orders of magnitude [24] . We thus expect two things when introducing the corresponding mutations K5A and L9A into αDTX-lumitoxins. First, we expect the initial K + current to increase, as our model predicts that decreasing the peptide affinity results in fewer channels being blocked in the dark (off) state. Second, we expect the activation ratio ( I lit / I dark ) to decrease as fewer channels are now primed to become unmasked by illumination. We experimentally confirmed these expectations, and, after investigation of a suite of mutated αDTX–lumitoxins ( Fig. 3a ), we found that both baseline current and activation ratio depended monotonically on peptide toxin affinity, as would be expected given previous reports on free, that is non-tethered, toxin [24] , and consistent with our predictions. For example, the mutations R3A and R4A, which decrease the binding affinity 10-fold for free αDTX, decreased the activation ratio by 20%. The mutations K5A and L9A, which decrease the binding affinity >1,000-fold, completely abolished the light-dependent increase in K + current ( Fig. 3b ). 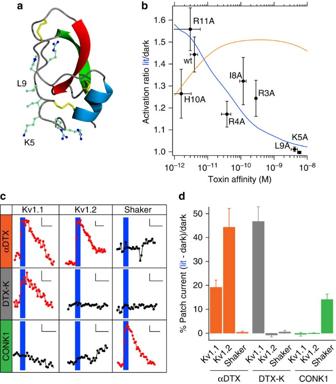Figure 3:Lumitoxin variants created through rational protein design can be incorporated into the modular lumitoxin architecture. (a) Mutated residues (shown as stick diagrams) mapped on the αDTX crystal structure (PDB accession number: 1DTX, shown as a cartoon). Residues labelled (K5, L9) are discussed in the text. (b) Average ratio of whole-cell K+current (Kv1.2 in PC12) during versus before illumination with 500 μW mm−2for αDTX variants as a function of reported toxin affinity24. Plotted throughout is the mean plus or minus s.e.m.,n=7–20 cells each point. Solid lines are simulated ratios assuming that mutations affect either solely the peptide toxin’s association rate constant α (blue line) or the dissociation rate constant β (orange line). (c) Representative current trace for indicated lumitoxin/channel combinations in response to illumination (blue bar). Inset scale bars: 50 pA (ordinate), 50 s (abscissa). (d) Lumitoxin-specific increase in whole-cell patch in response to illumination with blue light (500 μW mm−2) for specific Kv channels.n=3–20. Figure 3: Lumitoxin variants created through rational protein design can be incorporated into the modular lumitoxin architecture. ( a ) Mutated residues (shown as stick diagrams) mapped on the αDTX crystal structure (PDB accession number: 1DTX, shown as a cartoon). Residues labelled (K5, L9) are discussed in the text. ( b ) Average ratio of whole-cell K + current (Kv1.2 in PC12) during versus before illumination with 500 μW mm −2 for αDTX variants as a function of reported toxin affinity [24] . Plotted throughout is the mean plus or minus s.e.m., n =7–20 cells each point. Solid lines are simulated ratios assuming that mutations affect either solely the peptide toxin’s association rate constant α (blue line) or the dissociation rate constant β (orange line). ( c ) Representative current trace for indicated lumitoxin/channel combinations in response to illumination (blue bar). Inset scale bars: 50 pA (ordinate), 50 s (abscissa). ( d ) Lumitoxin-specific increase in whole-cell patch in response to illumination with blue light (500 μW mm −2 ) for specific Kv channels. n =3–20. Full size image We do not know whether mutations in αDTX affect the lumitoxin affinity through altering peptide toxin/channel association or dissociation. However, by using the model developed above, we can simulate the theoretical activation ratios of αDTX–lumitoxin variants using either assumption and found that the effects of all mutations except H10A on the experimentally determined activation ratios were consistent with a decrease in the association rate constant ( Fig. 3b , solid lines). Lumitoxins are modular and channel specificity is adjustable In the ideal case, it would be possible to tether multiple light-switchable protein ligands to the cell membrane without any optimization of the non-ligand protein parts. Consequently, we explored whether the lumitoxin architecture fulfills this requirement by creating lumitoxin genes containing different peptide toxins that target distinct Kv channel types. Whereas αDTX blocks both Kv1.1 and Kv1.2 channels [28] , Dendroaspis polylepis DTX-K, which shares only 63% sequence identity with αDTX, blocks mainly Kv1.1 channels [29] . Conkunitzin-S1 (CONK1), isolated from the marine cone snail Conus striatus , specifically blocks the Drosophila Shaker Kv channel [30] . We expressed the resulting lumitoxins in mammalian cell culture co-transfected with the Kv channels Kv1.1, Kv1.2 and Shaker. We used a variant of the Shaker Kv containing a mutation (K427D) shown to increase CONK1 affinity [30] . Whole-cell patch clamp electrophysiology reveals a clear specificity in the ability of lumitoxins to modulate K + currents in response to blue-light illumination (500 μW mm −2 ). Whereas αDTX-containing lumitoxins affect both Kv1.1 and Kv1.2, but not Shaker (K427D) ( Fig. 3c upper row, Fig. 3d ), DTX-K-containing lumitoxins are specific for Kv1.1 ( Fig. 3c middle row, Fig. 3d ). Similarly, CONK1-containing lumitoxins only affect Shaker Kv channels, but not the mammalian homologs Kv1.1 or Kv1.2 ( Fig. 3c bottom row, Fig. 3d ). These results imply that lumitoxin specificity can be altered by swapping the genetically encoded protein ligand without the necessity of optimizing non-ligand protein domains, resulting in multiple genetically encoded reagents for the actuation of specific subclasses of endogenous Kv channels. We here present the architecture of a fully genetically encoded tool for modulating the concentration of a protein ligand near the surface of a specified cell or set of cells by light. The resultant ‘lumitoxins’ are fusion proteins of two fundamentally useful functional elements, peptide neurotoxins and the photoreceptor LOV2-Jα, which serves as the tether between the protein ligand and the membrane. We demonstrated the functionality of our technology by creating several genetically encoded peptide toxins, targeting different classes of Kv channels, whose concentration could be modulated by light, in a fully reversible manner. Our architecture was capable of yielding lumitoxins that modulated K + currents with subfamily precision (for example, favouring Kv1.1 over Kv1.2 with perfect discrimination), demonstrating that peptide toxins, when part of a light-activated membrane-tether fusion protein, retain their activity and specificity. This specificity might be further facilitated by the addition of subcellular protein-trafficking motifs so that, for example, just the subset of Kv channels located on the axons or dendrites might be modulated. Exploring whether other classes of ion channels, and other membrane proteins such as neurotransmitter receptors, GPCRs, receptor tyrosine kinases and so forth, can be actuated by lumitoxins may represent a natural field of exploration in the future. In earlier studies, the LOV domain had been customized in several ways to embed various different peptides and enzymes within or next to the LOV domain [31] , [32] , [33] . Our new architecture is modular in the sense that the LOV domain does not require customization for each target peptide and thus might present a more general solution to make peptides or proteins available upon illumination. Another set of earlier studies fused protein ligands to membrane anchors, enabling fully genetically encoded blockade of endogenous ion channels [9] , [10] , [11] . Our architecture builds on these pioneering studies by enabling ion channel activity to be dynamically controlled over rapid timescales. Finally, a third line of past inquiry utilizes light-responsive, externally added chemical ligands anchored to specific sites engineered into ion channels [13] , [14] , [15] , [16] , [17] , [18] , [19] , enabling fast induction and reversal, by modulating the concentration of the ligand relative to the ion channel surface. Our current methodology extends these ideas by being fully genetically encoded, eliminating the need for exogenous chemical application. We developed an analytical model for lumitoxin function, based on biophysical principles, and focusing on the hypothesis that the illumination of the lumitoxin would, as the LOV2-Jα unfolds, modulate the local concentration of the peptide toxin near the cell surface when expressed on cellular membranes. In our theory, the signal magnitude is not determined by the detailed interactions between the LOV2 domain and the coupled effector domain (here, a peptide toxin), as in past LOV-based optogenetic tools [31] , [32] , [33] , [34] , but rather by the difference in length and rotational freedom of the Jα helix between lit and dark states, which directly influences the difference in local concentration near the cell surface. Both the apparent forward and backward rates of the αDTX-containing lumitoxin are similar to the unfolding and folding kinetics of the isolated AsLOV2 domain [26] , [27] , hinting at the rate-limiting step in light switching for lumitoxins utilizing AsLOV2 as the photoswitch. Our models, protein ligand swaps, and mutagenesis data suggest that the lumitoxin architecture is sufficiently modular for AsLOV2 properties such as kinetics, helix folding equilibrium, and so on to be engineered independent of protein ligand and anchor context, allowing for upgrades or altered performance of lumitoxins. Thus, our strategy represents a potentially important modular and tunable architecture in the field of engineered light-activated proteins. Note that, in this context, the high light sensitivity of lumitoxins (activated by as little as 10 μW mm −2 ) relative to ‘traditional’ optogenetic tools such as ChR2 (routinely driven by >1,000 μW mm −2 ) may enable lumitoxins to be incorporated into existing experimental contexts without requiring disturbance of other engineered signaling pathways. Systematic studies of a variety of different protein ligands, together with other structural features of lumitoxins such as linker length, composition and choice of membrane anchor, are needed to expand the family of lumitoxin reagents and improve its functional characteristic. Lumitoxins capable of blockading channels in response to light, in addition to mediating their actuation, would also be particularly useful. In the future, the lumitoxin architecture, or future variants thereof, might be utilized to tether arbitrary genetically encoded payloads beyond Kv channel modulating protein ligands—neuropeptides, growth factors, signaling domains—close to membrane-associated ion channels and receptors without requiring extensive re-optimization of the protein architecture. Modelling tethered-particle motion and lumitoxin stimulation A system of two spheres, representing a LOV2 domain (2 nm diameter) and a peptide toxin (0.75 nm diameter), connected to each other and a solid wall via linkers with a variable number of elements (0.2 nm diameter) representing linker amino acids, was simulated in MATLAB. Each linker element ( n ) was connected to its neighbouring linker elements (n+1 and n−1) with springs (spring constant 0.5 N m −1 ) at the distance of a peptide bond (0.4 nm). Pairs of second nearest neighbour elements were also connected to each other with a spring (spring constant 0.25 N m −1 ) in order to maintain the equilibrium bond angle between them at 109 degrees. Fluctuations of this system because of Brownian motion took the form and were simulated for 150 ns for several combinations of lengths of linkers. Modelling of lumitoxin stimulation was performed using MATLAB scripts numerically integrating a set of ordinary differential equations describing the thermodynamic model depicted in Fig. 1c . Simulation parameters were n (Toxin)= n (Channel)=8,000; reaction volume=3.2 × 10 −14 l (corresponding to a 13-μm (inner radius) hollow sphere with 15 nm wall thickness); α =2 × 10 8 M −1 s −1 ; α *=6.6 × 10 7 M −1 s −1 ; β =2 × 10 −2 s −1 ; k on (lit)=2.5 × 10 −1 s −1 , k on (dark)=1.6 × 10 −3 s −1 , k off =2.55 × 10 −2 s −1 . For theoretical activation ratios ( Fig. 3b ) α ranged from 5 × 10 4 to 4 × 10 8 M −1 s −1 , α * ranged from 1.7 × 10 4 to 1.4 × 10 8 M −1 s −1 , and β ranged from 2 × 10 −4 to 4 s −1 . Molecular biology and construct generation Genes encoding for fusion proteins were assembled as a multicomponent cloning cassette from annealed oligonucleotides (IDT DNA) containing these elements (in order): Bgl II or Nhe I—Secretion Signal/FLAG tag— Hin dIII—(αDTX or DTX-K or CONK1)— Kpn I—Linker—LOV2-Jα(404-546)— Not I—PDGF-R-mCherry— Xba I. PDGF-R-mCherry was derived from pFU-MVIIA-PC (Addgene) [10] . See Table 1 for sequence details. This cassette was inserted into the mammalian expression vector pcDNA3.1(+) (Invitrogen) using Nhe I/ Xba I restriction sites. The respective genes coding for rat Kv1.2 (Kv1.2), rat Kv1.1 (Kv1.1) or Shaker were amplified from Kv1.2-pBluescript, Shaker-pBluescript (gifts from Roderick Mackinnon), or BacMam Kv1.1 (Invitrogen) and inserted into pcDNA3.1(+) or pEGFP-N3 using Bam HI/ Eco RI or Nhe I/ Eco RI, respectively. Both αDTX–lumitoxin and Kv1.2 cassettes were also inserted into the bidirectional expression vector pBI-CMV1 (Clontech) using Bgl II/ Xba I and Bam HI/ Not I sites, respectively, to drive expression from the same plasmid. Table 1 Lumitoxin construct generation. Full size table Mammalian cell culture PC12 cells (ATCC) were maintained in DMEM (Cellgro), 10% fetal bovine serum (Invitrogen), 5% donor horse serum (Invitrogen), 1% penicillin/streptomycin (Cellgro) and 1% sodium pyruvate (Biowhittaker). For electrophysiological recordings and imaging, cells were plated on glass coverslips treated with Matrigel (BD Bioscience). Adherent cells were transfected usingLipofectamine LTX (Invitrogen) following the manufacturer’s instructions and recorded 36–48 h later. For confocal microscopy, cells were fixed with 4% formaldehyde, permeabilized with 0.4% saponin and either stained with anti-FLAG M2 peptide antibody (Sigma A2220, 1:1,000 dilution) followed by anti-mouse-Alexa488 secondary antibody staining (Invitrogen) or directly observed using mCherry fluorescence. Electrophysiology and illumination K + currents were recorded from PC12 cells 36–48 post-transfection using whole-cell voltage clamp. Analog signals were filtered (1–5 kHz) using the built-in 4-pole Bessel filter of an Axopatch 200B patch clamp amplifier (Molecular Devices), digitized at 10 kHz (Digidata 1440 A, Molecular Devices) and stored on a computer hard disk. The bath solution contained the following (mM): 125 NaCl, 2 KCl, 3 CaCl 2 , 1 MgCl 2 , 10 HEPES, 30 glucose, adjusted to pH 7.3 with NaOH. Electrodes were drawn from borosilicate patch glass (Warner Instruments) to a resistance of 5–10 MΩ. Patches with access resistance of >50 MΩ were discarded from the data analysis. The reported n refers to the number of patched cells. Cells were screened for mCherry expression using a 565-nm high-power LED (Thorlabs) filtered by a 560±40-nm bandpass filter (Semrock) through a 40 × lens. Lumitoxins were stimulated with a 455-nm high-power LED (Thorlabs). Accession codes: Construct sequences have been deposited in the DDBJ/EMBL/GenBank nucleotide database under accession codes KF878105 (aDTX-Lumitoxin), KF878106 (CONK1-Lumitoxin) and KF87810 (DTX-K-Lumitoxin) and are available on request at http://syntheticneurobiology.org/protocols . How to cite this article: Schmidt, D et al. A fully genetically encoded protein architecture for optical control of peptide ligand concentration. Nat. Commun. 5:3019 doi: 10.1038/ncomms4019 (2014).